Tenfold increase in the lifetime of blue phosphorescent organic light-emitting diodes Organic light-emitting diodes are a major driving force of the current information display revolution due to their low power consumption and potentially long operational lifetime. Although electrophosphorescent organic emitters have significantly lower power consumption than fluorescent emitters, the short lifetime of electrophosphorescent blue devices has prevented their application in displays for more than a decade. Here, we demonstrate a novel blue electrophosphorescent device with a graded dopant concentration profile in a broadened emissive layer, leading to a lower exciton density compared with a conventional device. Thus, triplet-polaron annihilation that leads to long-term luminescent degradation is suppressed, resulting in a more than threefold lifetime improvement. When this strategy is applied to a two-unit stacked device, we demonstrate a lifetime of 616±10 h (time to 80% of the 1,000 cd m −2 initial luminance) with chromaticity coordinates of [0.15, 0.29], representing a tenfold lifetime improvement over a conventional blue electrophosphorescent device. Organic light-emitting diodes [1] (OLEDs) are current-driven electroluminescent devices that have been proven successful in enabling a range of applications, including mobile displays, televisions and lighting [2] , [3] , [4] . Following electron-hole recombination, two types of molecular excited states (called excitons), singlets and triplets, are formed with a ratio of 1:3 determined by quantum spin statistics [5] . Fluorescent OLEDs employ spin-antisymmetric singlets for emission, and thus have the internal quantum efficiency (IQE) limit of 25%. Although triplet–triplet annihilation can be used to improve the IQE of fluorescent OLEDs beyond this limit [6] , [7] , their efficiencies are far inferior to the routinely realized 100% IQE [8] in electrophosphorescent OLEDs (PHOLEDs) [9] that use both singlets and spin-symmetric triplet states for emission. Besides high efficiency, long operational lifetime is essential for a technology to achieve commercial success. After more than a decade of research, significant breakthroughs in the lifetime of green and red PHOLEDs have been achieved, with reported T50 (time to 50% of the initial luminance L 0 =1,000 cd m −2 ) as long as 10 6 h [10] , [11] , [12] , [13] . Even longer lifetimes have been reported at manufacturers’ websites (see, for example, www.udcoled.com ). In contrast, surprisingly little progress has been made in the improvement of blue PHOLED lifetime. For example, a T50 of only several hours for L 0 =1,000 cd m −2 has been reported for a PHOLED with the blue emitting iridium (III) FIrpic (bis[(4,6-difluorophenyl)-pyridinato-N,C 2′ ] picolinate) [14] as the emitter [15] . As a result, relatively inefficient blue fluorescent OLEDs remain dominant in OLED displays, making the blue pixels a bottleneck to improvements in display performance. It has been suggested that the intrinsic degradation of blue PHOLEDs results from energetically driven formation of traps [16] , [17] that can quench excitons and also act as non-radiative charge recombination centres. These traps are formed due to bimolecular triplet-polaron annihilation (TPA) where energy is transferred from triplets to polarons (that is, charged molecules). This, in turn, results in a high-energy polaron (approximately twice the triplet energy) that, on thermalization, can break bonds on the molecule on which it resides. Owing to their high triplet energy, excess energy dissipated through TPA in blue PHOLEDs is significantly higher than for red or green PHOLEDs, explaining the faster degradation in the former case. Furthermore, although blue fluorescent devices are by no means immune to this degradation path, their lower triplet energies lead to lower energy dissipation, and thus less destructive TPA events. Since these fundamental mechanisms were first identified, to our knowledge there has been no direct evidence that blue PHOLED lifetime can be improved by reducing TPA in a practical, high-efficiency device. One potential route to reduce degradation suggested by this analysis is to decrease the exciton density in the emissive layer (EML) and consequently reduce the occurrence of TPA. Recently, Erickson and Holmes [18] have demonstrated increased efficiency by the extension of the exciton formation zone in a green PHOLED from 15 nm to >80 nm through graded mixing of electron and hole-transporting host molecules. No lifetime data were reported in that work. In addition, the use of a non-uniform dopant profile in OLEDs was previously reported [19] , [20] , [21] to improve efficiency; however, it is unclear whether the PHOLED exciton formation zone was also broadened as a consequence of the profiles employed, and its consequences on device lifetime were not explored. Here we show that grading the blue dopant in the EML of a PHOLED significantly extends the lifetime of the device by extending the exciton formation zone. The broadening of the exciton distribution, and hence the device lifetime, is further increased by using a sufficiently high concentration of a dopant whose highest occupied molecular orbital level (HOMO) is chosen above that of the host to allow for holes to conduct directly on the dopant. To our knowledge, this is the first report of an OLED with a graded doping profile that extends the distribution of excitons within the EML, thus significantly having an impact on device operational lifetime. Furthermore, engineering the dopant and host frontier energy levels in addition to concentration grading provides a powerful tool that can be used to develop materials systems and device architectures to extend device lifetime even beyond that reported here. 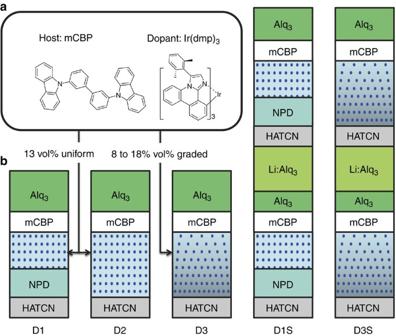Figure 1: Structures of the blue PHOLEDs. (a) Chemical structures of the host mCBP and phosphorescent dopant Ir(dmp)3used in the EMLs of the blue PHOLEDs. (b) PHOLED device structures. HATCN, NPD and Alq3are used for the HIL, HTL and electron transport layer (ETL) materials, respectively. The EMLs of both D1 and D2 employ a 13 vol% doping concentration, and D2 replaces the HTL in D1 with an EML. D3 has an EML with the doping concentration graded from 18 to 8 vol% with a maximum at the EML/HIL interface. Further, D1S and D3S are two-unit stacked OLEDs with 2 vol% Li-doped Alq3and HATCN as the interconnecting layers. PHOLED device structure and characteristics Figure 1a shows the chemical structure of the host 4,4′-bis(3-methylcarbazol-9-yl)-2,2′-biphenyl (mCBP) and blue dopant iridium (III) tris[3-(2,6-dimethylphenyl)-7-methylimidazo[1,2-f] phenanthridine] (Ir(dmp) 3 ) [17] . We compare five PHOLEDs shown in Fig. 1b , with their structural details provided in Methods. The hole transport layers (HTLs) and/or EMLs of the devices D1–D3 consist of a 20-nm-thick layer of 4,4′-bis[N-(1-naphthyl)-N-phenyl-amino]-biphenyl and a 30-nm-thick 13 vol% Ir(dmp) 3 doped in mCBP (Device D1), 50-nm-thick 13 vol% Ir(dmp) 3 doped mCBP (Device D2) and a 50-nm layer of Ir(dmp) 3 doped mCBP, with the doping concentration varying linearly with position (Device D3) from 18 vol% (close to the anode) to 8 vol% (close to the cathode). Devices D1S and D3S are two-unit stacked OLEDs whose HTL/EMLs are analogous to D1 and D3, respectively. Here, D1 adopts a conventional OLED structure almost identical to the blue PHOLED reported previously [17] and serves as the control device. Figure 1: Structures of the blue PHOLEDs. ( a ) Chemical structures of the host mCBP and phosphorescent dopant Ir(dmp) 3 used in the EMLs of the blue PHOLEDs. ( b ) PHOLED device structures. HATCN, NPD and Alq 3 are used for the HIL, HTL and electron transport layer (ETL) materials, respectively. The EMLs of both D1 and D2 employ a 13 vol% doping concentration, and D2 replaces the HTL in D1 with an EML. D3 has an EML with the doping concentration graded from 18 to 8 vol% with a maximum at the EML/HIL interface. Further, D1S and D3S are two-unit stacked OLEDs with 2 vol% Li-doped Alq 3 and HATCN as the interconnecting layers. Full size image The current density–voltage–luminance ( J–V–L ), external quantum efficiency (EQE) and emission spectral characteristics of the five devices are shown in Fig. 2 and are summarized in Table 1 . Replacing the HTL in D1 with an EML in D2 results in an increase in the operating voltage, as expected. Moreover, the use of a graded doping profile in the EML (D3) decreases the voltage compared with the uniformly doped D2. The EQE of D1 and D2 are almost identical above 1 mA cm −2 , whereas the EQE of D3 is >10% higher than those of D1 and D2. As expected [22] , D3S has approximately double the voltage and EQE compared with D3; for example, at 10 mA cm −2 , D3S operates at a voltage of 17.4 V and EQE=17.2% compared with 8.5 V and 9.3% for D3. Similar trends also exist between D1 and D1S. The spectra of D1, D2, D3 and D3S are almost identical, although the D1S spectrum shows a slightly higher vibronic peak energy at ~500 nm, due to optical microcavity effects [23] . 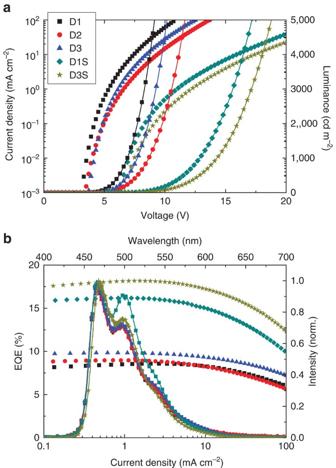Figure 2: Performance characteristics of the blue PHOLEDs. (a) Current density–voltage (J–V, scattered markers) and luminance–voltage (L–V, line-connected markers) characteristics. (b) EQE versusJ(left axis) and emission spectra (right axis). Figure 2: Performance characteristics of the blue PHOLEDs. ( a ) Current density–voltage ( J–V , scattered markers) and luminance–voltage ( L–V , line-connected markers) characteristics. ( b ) EQE versus J (left axis) and emission spectra (right axis). Full size image Table 1 Characteristics at L 0 =1,000 cd m −2 and lifetime fitting parameters for blue emitting PHOLEDs. * Full size table Charge transport and recombination To understand the charge transport characteristics in the EML, we measured the ultraviolet photoelectron spectra of thin films of mCBP, Ir(dmp) 3 , as well as Ir(dmp) 3 deposited on mCBP (see Supplementary Figure 1 ). After considering the dipole energy shift when Ir(dmp) 3 is deposited on mCBP, then mCBP and Ir(dmp) 3 have HOMO energies of 6.0 and 5.0 eV, respectively, as illustrated in Fig. 3a . Thus, it is expected that at sufficiently high concentrations, the dopant supports hole transport in the EML. The conduction mechanism is confirmed by the J–V characteristics of hole-only devices that show improved hole transport when increasing the Ir(dmp) 3 concentration in mCBP, as reported in Supplementary Figure 2 . Also shown in Supplementary Figure 2 are the conduction characteristics of electron-only devices, which indicate electron transport in the EML occurs solely through mCBP. 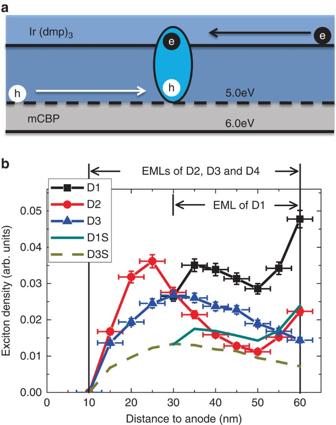Figure 3: Energetics and exciton density profiles in the PHOLED EML. (a) Electron and hole transport and recombination energetics in the blue PHOLED EMLs. (b) Exciton density profile in the EMLs of D1–D3 calculated from ‘probe’ devices employing PQIr in the red light-emitting sensing layer. The profiles are normalized to integrated exciton densities in the EMLs of unity. Moreover, the exciton density profiles of D1S and D3S are calculated from the D1 and D3 profiles, respectively. The errors in distance to anode arise from the determination of the Förster transfer radius for Ir(dmp)3to PQIr of ~3 nm, and the errors in exciton density arise from the errors in EQEs (see Methods). Figure 3: Energetics and exciton density profiles in the PHOLED EML. ( a ) Electron and hole transport and recombination energetics in the blue PHOLED EMLs. ( b ) Exciton density profile in the EMLs of D1–D3 calculated from ‘probe’ devices employing PQIr in the red light-emitting sensing layer. The profiles are normalized to integrated exciton densities in the EMLs of unity. Moreover, the exciton density profiles of D1S and D3S are calculated from the D1 and D3 profiles, respectively. The errors in distance to anode arise from the determination of the Förster transfer radius for Ir(dmp) 3 to PQIr of ~3 nm, and the errors in exciton density arise from the errors in EQEs (see Methods). Full size image In this novel architecture, as illustrated in Fig. 3a , recombination occurs between an electron in the lowest unoccupied molecular orbital of mCBP and a hole in the Ir(dmp) 3 HOMO, resulting in an exciplex. As the PHOLED emission is solely from the phosphorescence of Ir(dmp) 3 , the intermediate exciplex state rapidly transfers its energy to the Ir(dmp) 3 triplet. Note that the thermalization loss when an electron on mCBP recombines with a hole in the Ir(dmp) 3 HOMO is 1.0 eV less than for a hole in the mCBP HOMO, contributing to the relatively high operational stability of the blue PHOLEDs. The hole conductivity in the graded EML of D3 increases as the distance to the hole injection layer (HIL)/EML interface is decreased due to the increasing concentration of Ir(dmp) 3 . In the opposite direction towards the EML/hole-blocking layer (HBL) interface, the hole conductivity decreases while the electron conductivity stays approximately constant. Thus, in contrast to the abrupt hole blocking by the EML/HBL interface in D1 and D2, in D3 the holes are gradually blocked by the hole conductivity gradient, leading to a simplified device architecture where the HTL is replaced by a high concentration of the hole-conducting phosphorescent dopant near the HIL. As a consequence, exciton formation in D3 occurs over an extended distance compared with either D1 or D2. Exciton distribution in the emission zone To determine the hole-blocking efficiency and thus the shape of the exciton formation zones in D1–D3, we fabricated a series of PHOLEDs with a thin, red-emitting ‘sensing’ layer using the red dopant, iridium (III) bis(2-phenyl quinolyl-N,C 2′ ) acetylacetonate (PQIr) whose relative emission intensity can provide information about the spatial distribution of excitons in the EML (see Methods). Here, PQIr is co-doped at 2 vol% at different positions separated by 5 nm in the EMLs of D1–D3, with a doping layer width of 1.5 nm. The HOMO and lowest unoccupied molecular orbital energies of PQIr are at 5.0 and 2.7 eV relative to the vacuum level, respectively [24] . Owing to the low doping concentration and narrowness of the sensing layers, their presence should not significantly affect the charge transport or recombination properties in the EML. This is confirmed by the almost identical J–V characteristics between devices with and without sensing layers (see Supplementary Figures 3, 4 and 5 for more details on the sensing layers). From the emission spectra and EQE at 10 mA cm −2 , as well as from the calculated light out-coupling efficiencies [25] in the ‘sensing’ PHOLEDs (see Methods and Supplementary Note 3 ), we calculate the exciton densities versus position in the EMLs of D1–D3, with results in Fig. 3b . In D1 (that is, the conventional blue PHOLED), significant exciton accumulation occurs at the EML/HBL interface. In D2 that lacks an HTL, the exciton formation zone is broadened due to the increase in the EML thickness. As a result, the exciton density at the HIL/EML interface is reduced due to a correspondingly low concentration of holes. However, because of the reduced hole-transport efficiency, electrons penetrate deep into the EML, resulting in a peak exciton density near the HIL/EML interface. In contrast, efficient hole transport near the HIL/EML interface and the gradual hole blocking in the EML in D3 lead to a more uniform exciton distribution (and hence higher EQE) compared with both D1 and D2, with a peak density near to the centre of the EML. As the EMLs of D1 and D1S are identical, and D3 and D3S are also identical, Fig. 3b also shows exciton density profiles of D1S and D3S, estimated at 50% of the exciton density in D1 and D3 due to the almost doubled EQEs. 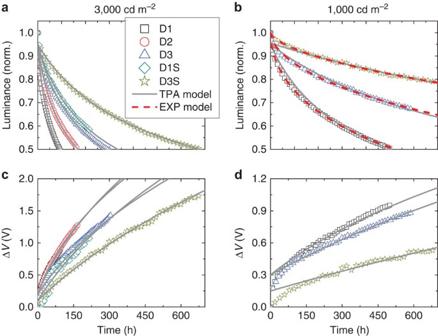Figure 4: Operational lifetime of the PHOLEDs. Time evolution of the normalized luminance,L, of blue PHOLEDs and change in operating voltage ΔV(offset to zero) at the initial luminance ofL0=3,000 cd m−2(a,b) and 1,000 cd m−2(c,d). The data are fit to the TPA model using the exciton density profiles inFig. 3b. The luminance forL0=1,000 cd m−2(c) are also fit to the adjusted empirical exponential (EXP) model to estimateT50(that is, degradation time leading to 50% decrease inL). PHOLED lifetime: experiment and model Figure 4 shows the time evolution of the luminance, L , and the change in voltage from its initial value, ΔV =| V(t=0)−V(t) |, for D1, D3 and D3S tested at room temperature and a constant current density for two initial luminances: L 0 =1,000 and 3,000 cd m −2 . In addition, we show these same characteristics for D2 and D1S tested at L 0 =3,000 cd m −2 . The lifetimes show an increasing trend from D1 through D3, with T80 =11.5, 24.5 and 39 h, respectively, for D1–D3 at L 0 =3,000 cd m −2 , consistent with the broadened exciton formation zone of the latter two devices ( Fig. 3b ). Note that T80 for the control, D1, is consistent with similar results for this device reported previously [6] , and is only ~29% that of the graded device, D3. Further, due to the reduced triplet density in the stacked OLEDs, T80 =48 and 106 h for D1S and D3S, respectively. At L 0 =1,000 cd m −2 , T80 =616±10 h for D3S, representing >10 times improvement from the previously investigated [17] control, D1. The improvement in T50 for D3S is slightly less significant than T80 , leading to an approximately sevenfold increase from D1. Figure 4: Operational lifetime of the PHOLEDs. Time evolution of the normalized luminance, L , of blue PHOLEDs and change in operating voltage Δ V (offset to zero) at the initial luminance of L 0 =3,000 cd m −2 ( a , b ) and 1,000 cd m −2 ( c , d ). The data are fit to the TPA model using the exciton density profiles in Fig. 3b . The luminance for L 0 =1,000 cd m −2 ( c ) are also fit to the adjusted empirical exponential (EXP) model to estimate T50 (that is, degradation time leading to 50% decrease in L ). Full size image To establish a quantitative relationship between the exciton density profiles and operational lifetimes, we model L and ΔV as functions of time, t , using a model similar to Giebink et al . [17] (see Methods). Briefly, the degradation of both L and V are attributed to the formation of traps in the EMLs due to TPA at a rate, k Q . The following trap bimolecular interactions are considered: trap–electron interactions at rate [17] , k Qn =1.44 × 10 −13 cm 3 s −1 ; trap–hole interactions at rate [17] , k Qp =4.8 × 10 −14 cm 3 s −1 ; and trap–triplet annihilation at rate, k QN . Trap formation depends on the local exciton density; hence, we model PHOLED degradation using the profiles in Fig. 3b . The model is fit to the degradation characteristics of all devices with k Q and k QN as free parameters (see Table 1 ); all other parameters are as previously determined for this materials combination [17] (see Methods). Yamamoto et al . [26] reported that water contamination of organic films during deposition leads to an accelerated initial degradation when the deposition background pressure is >5 × 10 −8 Torr for PHOLEDs, almost identical to that of D1. In our case, organic films were deposited in a system with a base pressure of 5 × 10 −7 Torr; however, the TPA model ignores extrinsic effects such as water contamination. To account for these effects in our fits, t =0 corresponds to a normalized luminance of 0.95 and the initial value of ΔV was chosen to be non-zero (see Methods). From the lifetime fit parameters summarized in Table 1 , k Q and k QN in all five devices are almost identical, indicating that the differences in their lifetimes are quantitatively explained by their different exciton densities at the same luminance. Compared with D1, the doubled lifetime in D2 is simply a result of changes in the exciton density profile, and the tripled lifetime in D3 is due to the increase in EQE (leading to a decrease of J to achieve a given L 0 ), as well as to the significant spreading of the exciton formation zone. Here, the novel graded doping profile in a thick EML results in a threefold improvement in lifetime compared with the conventional uniform doping profile in a thin EML. At 3,000 cd m −2 , the improvement in T80 from single element to stacked OLEDs is 4.1-fold from D1 to D1S, and 2.7-fold from D3 to D3S. This is understandable from the decrease in J (and thus triplet densities); at 3,000 cd m −2 , J of D1S is 42% of D1, and J of D3S is 52% of D3. The more significant decrease in J in D1S is due to the increase of its spectral peak at 500 nm (see Fig. 2b ), which results in a higher luminance efficiency (in cd A −1 ) at the same EQE. Thus, when combining the graded doping profile with a stacked structure, a tenfold improvement in T80 from D1 to D3S is observed. Note that the TPA model considers degradation in the thin film bulk, but not at the interface [27] . Indeed, the low exciton density at the EML/HBL interface in D3 and D3S may also contribute to the observed increase in lifetime by reducing the rate of damage at this interface. To estimate T50 at L 0 =1,000 cd m −2 for D3 and D3S, we extrapolate the TPA model fits. In addition, an empirical method often employed to model OLED degradation uses the adjusted exponential decay function: [28] . Here, τ and β are phenomenological parameters. This model also results in reasonable fits to the degradation data ( Fig. 4c ) and provides extrapolated values for T50 similar to those obtained from the physics-based TPA model ( Table 1 ). From these fits, T50 =3,500 h at L 0 =1,000 cd m −2 for D3S, which approaches that of blue fluorescent OLEDs with T50 ~10 4 h (see, for example, www.idemitsu.com ). Note that the emission of the devices reported here is light blue (although more saturated than the cyan colour of FIrpic). Colour tuning to achieve more saturated blue emission is commonly achieved in fluorescent blue display sub-pixels through the use of microcavities [23] , [29] and/or colour filters. For example, a 70-nm-thick anode of indium-tin oxide (ITO) yields Commission Internationale d’Eclairage chromaticity coordinates of [0.16, 0.26] [26] , compared with [0.16, 0.31] for a 120-nm-thick ITO layer due to weak microcavity effects (see Supplementary Figure 6 ). Although the blue PHOLED lifetime reported here remains substantially less than that of red and green PHOLEDs at similar luminances, blue sub-pixels in displays operate at a considerably lower luminance than either the red or green sub-pixels. For example, the required luminance to achieve an sRGB colour gamut [30] for green is 9.9 times the luminance for blue. Thus, a comparison between blue and green PHOLED lifetimes for displays suggests that the blue PHOLED sub-pixel luminance needs to be only ~10% that of the green. Under such conditions (that is, L 0 =100 cd m −2 ), the TPA model estimates the blue PHOLED lifetime is 70,000 h. Moreover, adopting a degradation acceleration factor that relates luminance to lifetime [28] , viz . with n =1.55, the extrapolated blue PHOLED lifetime is 1.3 × 10 5 h. These lifetimes approach the commercial green PHOLED lifetime (10 6 h) at L 0 =1,000 cd m −2 . In summary, we demonstrate a tenfold increase in blue PHOLED lifetime employing a stacked PHOLED structure with two EMLs having graded phosphorescent dopant concentrations. Grading used in combination with engineered frontier orbital energies of both the dopant and host materials significantly decreases the exciton density across the emission zone. This in turn increases the blue PHOLED external efficiency while reducing detrimental TPA that decreases device lifetime. Considering the different colour sub-pixel luminances used in displays, the improved blue PHOLED lifetimes approaches that of green PHOLEDs under normal operating conditions. The novel device architecture employed is based on a fundamental physical understanding of the relationship between energy-driven TPA and device degradation, and hence should be generally applicable to a wide range of phosphorescent and fluorescent devices. Further lifetime improvements are anticipated by finding dopant/host combinations with conduction properties similar to the materials used here, and which minimize interactions between triplets on the dopant and polarons on the host molecules that lead to molecular decomposition. Device fabrication Thin films were deposited by thermal evaporation on pre-cleaned ITO-on-glass substrates in a system with a background pressure of ~5 × 10 −7 Torr. Devices D1–D3 have the following structure: 120 nm ITO anode/10 nm hexaazatriphenylene hexacarbonitrile (HATCN) HIL/50 nm HTL+EML/5 nm mCBP HBL/30 nm tris(8-hydroxyquinolinato)aluminum (Alq 3 ) electron transport layer/1.5 nm 8-hydroxyquinolinato lithium (Liq)/100 nm Al cathode. The structure of D1S and D3S is 120 nm ITO/10 nm HATCN/50 nm HTL+EML/5 nm mCBP/5 nm Alq 3 /70 nm 2 vol% Li-doped Alq 3 /10 nm HATCN/50 nm HTL+EML/5 nm mCBP/25 nm Alq 3 /1.5 nm Liq/100 nm Al. All devices were grown on pre-patterned ITO with an active area of 2 mm 2 defined by openings in a polyimide layer that define the pixels. The PHOLEDs are packaged in an ultra-high purity N 2 -filled glove box with <0.5 p.p.m. oxygen and water concentration without exposure to air, following film deposition, by attaching a glass lid to the substrate using an epoxy seal around the perimeter. Devices for exciton sensing were grown on 70 nm of ITO with an active area of 0.785 mm 2 defined by shadow masks during cathode deposition. Device characterization J–V–L characteristics were measured using a parameter analyser (HP4145, Hewlett-Packard) and a calibrated photodiode (FDS1010-CAL from Thorlabs) following standard procedures [31] . Emission spectra were measured with a calibrated fibre-coupled spectrometer (USB4000, Ocean Optics) at J =10 mA cm −2 . Lifetime tests were carried out with PHOLEDs driven by constant current sources (U2722, Agilent), and the voltage and luminance are recorded by a data logger (Agilent 34972A). Exciton formation zone analysis Local exciton densities N(x) in the EMLs are calculated from the measured emission spectra, EQE (x) and the calculated outcoupling efficiency η R ( x ) (at a wavelength of 595 nm corresponding to the peak in the PQIr emission spectrum), from PHOLEDs with PQIr sensing layer at position x using: Here, A is a normalization factor such that , is the outcoupled photon number ratio from PQIr versus Ir(dmp) 3 , obtained from the ratio of red and blue peaks of the emission spectra. Degradation model The time evolution of L(t) and V(t) is modelled following Giebink et al . [17] by assuming trap (with density Q(x, t) ) formation due to TPA, and subsequent interactions with electrons with density n(x, t) , holes with density p(x, t) and excitons with density N(x, t) : Here r =1.7 × 10 −13 cm 3 s −1 is the Langevin recombination rate, τ N =1.1 μs is the triplet lifetime and G(x) is the local recombination rate, calculated from the local exciton density N(x) using , where e is the electron charge. Current densities at L 0 =1,000 cd m −2 are provided in Table 1 and at 3,000 cd m −2 are J= 21, 21, 17.5, 8.9 and 9.1 mA cm −2 for D1, D2, D3, D1S and D3S, respectively. Trap formation is attributed to TPA using: Then where B is a normalization factor, η B ( x ) is the calculated outcoupling efficiency at the peak emission wavelength of 466 nm for Ir(dmp) 3 , ε =3 is the relative permittivity and ε 0 is the vacuum permittivity. To account for the effect of water contamination during device fabrication [26] , L(0) is normalized to 0.95 and Δ V (0)=0.2 V (at 3,000 cd m −2 ) and 0.3 V (at 1,000 cd m −2 ) for D1–D3, and 0.1 V (at 3,000 cd m −2 ) and 0.15 V (at 1,000 cd m −2 ) for D1S and D3S. How to cite this article: Zhang, Y. et al . Tenfold increase in the lifetime of blue phosphorescent organic light-emitting diodes. Nat. Commun. 5:5008 doi: 10.1038/ncomms6008 (2014).